Unveiling thermal transitions of polymers in subnanometre pores The thermal transitions of confined polymers are important for the application of polymers in molecular scale devices and advanced nanotechnology. However, thermal transitions of ultrathin polymer assemblies confined in subnanometre spaces are poorly understood. In this study, we show that incorporation of polyethylene glycol (PEG) into nanochannels of porous coordination polymers (PCPs) enabled observation of thermal transitions of the chain assemblies by differential scanning calorimetry. The pore size and surface functionality of PCPs can be tailored to study the transition behaviour of confined polymers. The transition temperature of PEG in PCPs was determined by manipulating the pore size and the pore–polymer interactions. It is also striking that the transition temperature of the confined PEG decreased as the molecular weight of PEG increased. There is considerable current interest in the properties of polymers confined in nanometre scale spaces from both fundamental and practical perspectives. Nanofabrication processes have emerged on the basis of polymer nanoimprinting and wiring, so, it is essential to study the thermal stability of nanometre scale polymer assemblies over a wide range of temperatures; heat treatment induces structural decay or even collapse of polymer assemblies if this process is not carefully controlled [1] , [2] . Imprisonment of polymers in nanometre-sized channels is also important for transport and fluidic applications [3] , but thermodynamic responses of polymers are unexpectedly changed under these spatial constraints, limiting their practical use in nanodevices. In nanoconfined systems, the complication of polymer behaviour is a result of drastic changes in thermal transitions, such as melting–freezing and glass transitions, compared with those observed in bulk systems. Therefore, there is interest in gaining a quantitative understanding of confinement effects on the polymer thermal transitions occurring in the presence of finite size, surface forces and reduced dimensionality [4] , [5] , [6] , [7] , [8] , [9] , [10] , [11] , [12] . Thin film polymers [4] , [5] , [6] , [7] , nanocomposites [8] , [9] and porous matrices (for example, porous glass and clays) [10] , [11] , [12] have had dominant roles in elucidating the thermal transitions of polymer nanoassemblies. These previous systems have revealed the behaviour of confined polymers in several nanometre-to-micrometer range, but thermal transitions of polymers confined in subnanometre spaces (<1 nm), where only a few chains can exist, remained unexplored. For future applications of single- or few-chain polymers in molecular scale devices and advanced nanotechnology [13] , [14] , the study of thermal transitions in ultrathin polymer assemblies is highly desirable. In such constrained geometries, the conventional thermodynamics model becomes invalid, and specific polymer conformation and interface interactions may strongly affect thermal transitions [15] , [16] , which will offer an opportunity for detecting unprecedented behaviours in the confined polymer assemblies. Recent extensive research into the design and synthesis of porous coordination polymers (PCPs), prepared by the self-assembling process of metal ions and bridging organic ligands, has led to numerous practical and conceptual developments [17] , [18] , [19] , [20] . The characteristic features of PCPs are their high regularity, robustness and their precisely controllable channel structures with approximate molecular dimensions of 0.4–2 nm, which differ from those of conventional porous materials [20] . Thus, the regulated and tailor-made pore characteristics of PCPs are of key importance for achieving precision analysis of polymer confinement [21] , [22] . Taking advantage of PCPs, we can attain precision assembly of polymer chains within regular channels by controlling the thickness of chain bundles as well as tuning the environments of the chains. In this study, we report the first observation of cooperative thermal transition behaviour for systems containing only a few polymer chains confined in subnanometre-sized channels of PCPs, and demonstrate that multiple parameters of PCPs, such as pore size and surface functionality, determine the confinement effects on the polymer dynamics, resulting in systematic control of thermal transitions. [Cu 2 (L) 2 (ted)] n ( 1 ; L=dicarboxylates, ted=triethylenediamine) with one-dimensional (1-D) regular channels along the c -axis ( Fig. 1 and Supplementary Fig. S1 ) were employed as the host PCPs because their channel structures can be tuned by changing the dicarboxylate ligands, L [23] . A linear and crystalline polymer, polyethylene glycol (PEG; thickness of PEG chain=0.37 nm), was incorporated into the channels to probe confinement effects. 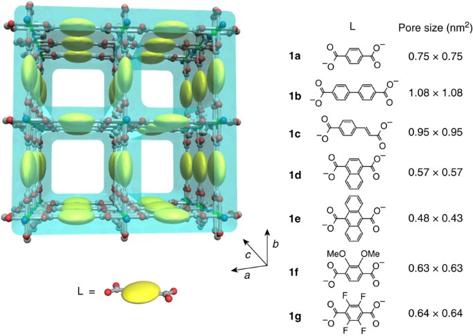Figure 1: Schematic image for nanochannel structures of PCP hosts. [Cu2(L)2(ted)]n(ted=triethylenediamine;1a, L=terephthalate;1b, L=biphenyl-4,4′-dicarboxylate;1c, L=styrenedicarboxylate;1d, L=1,4-naphthalenedicarboxylate;1e, L=9,10-anthracenedicarboxylate;1f, L=2,3-dimethoxy-1,4-benzenedicarboxylate; and1g, L=2,3,5,6-tetrafluoro-1,4-benzenedicarboxylate). Figure 1: Schematic image for nanochannel structures of PCP hosts. [Cu 2 (L) 2 (ted)] n (ted=triethylenediamine; 1a , L=terephthalate; 1b , L=biphenyl-4,4′-dicarboxylate; 1c , L=styrenedicarboxylate; 1d , L=1,4-naphthalenedicarboxylate; 1e , L=9,10-anthracenedicarboxylate; 1f , L=2,3-dimethoxy-1,4-benzenedicarboxylate; and 1g , L=2,3,5,6-tetrafluoro-1,4-benzenedicarboxylate). Full size image Characterization of PEG confined in PCP channels PEG with a very narrow molecular weight distribution ( M w =600, M w / M n =1.05) was introduced into [Cu 2 (terephthalate) 2 (ted)] n ( 1a ; channel size=0.75 × 0.75 nm 2 ), where the weight ratio of PEG to 1a was 0.4:1. This host can easily adsorb PEG in the channels to form a host–guest adduct ( 1a ⊃ PEG) with maintaining the framework structure via polymer melt processing [10] , [12] . Formation of the host–guest composite between 1a and PEG was fully confirmed by elemental analysis, X-ray powder diffraction (XRPD; Supplementary Fig. S2 ), scanning electron microscopy (SEM; Supplementary Fig. S3 ), particle size analysis ( Supplementary Fig. S4 ), nitrogen adsorption ( Supplementary Fig. S5 ) and various spectroscopic measurements ( Supplementary Figs S6–S10 ). All the obtained data support the complete encapsulation of PEG chains in the channels of 1a , and show no leakage of PEG from the host channels. The molecular conformation of PEG encapsulated in 1a was studied by conventional infrared measurements ( Supplementary Figs S8 and S9 ). The infrared bands of 1a ⊃ PEG detected at 915 and 950 cm −1 suggest the existence of a trans – trans – gauche conformation (– t O– t C– g C–) for the PEG chains [24] . This conformation is the most common structure of PEG and is usually observed in the bulk crystalline state [25] . However, in addition to these bands, the infrared spectrum of 1a ⊃ PEG showed clear peaks at 1,250 and 1,300 cm −1 , indicating that the PEG chains form a more linear structure with increasing trans conformation in the channels of 1a [24] . This stretched conformation of PEG would result from the confinement effect of 1a , in which the PEG chains are forced to form an extended linear structure in the narrow 1-D channels. 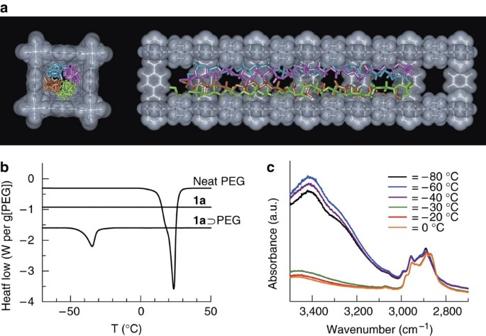Figure 2: Structure and thermal transition behaviour of PEG encapsulated in1a. (a) Typical MD structure of PEG 14-mer (Mw=634.7) encapsulated in the subnanometre channel. (b) DSC heating curves of neat PEG,1aand1a⊃PEG. (c) Variable temperature infrared spectra of1a⊃PEG.Mwof PEG used in these measurements was 600. Figure 2a shows the molecular dynamics (MD) structure of PEG confined in the channel of 1a . The conformation of the confined PEG seems almost linear and is different from the helical conformation of PEG chains in the bulk crystal [25] , which is fairly consistent with the results of infrared spectroscopies ( Supplementary Figs S8–S10 ). In this system, four PEG chains are maximally incorporated in the channel and are assembled with the linearly extended structure, with a slightly twisted conformation. Figure 2: Structure and thermal transition behaviour of PEG encapsulated in 1a . ( a ) Typical MD structure of PEG 14-mer ( M w =634.7) encapsulated in the subnanometre channel. ( b ) DSC heating curves of neat PEG, 1a and 1a ⊃ PEG. ( c ) Variable temperature infrared spectra of 1a ⊃ PEG. M w of PEG used in these measurements was 600. Full size image Thermal transition behaviour of confined PEG To investigate the thermal transition properties of PEG, differential scanning calorimetry (DSC) measurements were performed with neat PEG, 1a and 1a ⊃ PEG ( Fig. 2b ). The DSC scan for the neat PEG sample presented an endothermic peak at 22 °C for a melting temperature of PEG, and no transition was observed for the only host in this entire temperature region. In contrast, 1a ⊃ PEG clearly exhibited a transition at −36 °C, which is considerably lower than the melting temperature of neat PEG. Generally, DSC is not sensitive enough to detect any weak transitions of intercalated polymers and polymer composites with a low volume fraction [12] , [26] ; thus, any thermal transitions of PEG are not detected in the other porous materials with similar pore dimensions, for example, activated carbon fibre (ACF A-5; pore width=0.75 nm) and NaX zeolite (zeolite F-9; pore size=0.74 nm; Supplementary Fig. S11 ), because of irregular local topology and/or unsuitable chemical surfaces. Variable temperature infrared measurements of 1a ⊃ PEG indicated that the endothermic peak observed in the DSC scan corresponds to a transition of PEG itself confined in the channels ( Fig. 2c ). In the infrared spectra obtained at −80 to −40 °C, a broad peak assignable to the terminal OH group of PEG was found around 3,400 cm −1 , showing intermolecular hydrogen bondings among the PEG chains. This strong peak weakened upon warming the sample above −30 °C, together with a small peak shift of the C–H vibration of PEG from 2,890 to 2,869 cm −1 , which is similar to peak changes that are observed in neat PEG during its melting process [27] . In respect of the host framework, XRPD patterns of 1a ⊃ PEG with heating from −80 to 20 °C did not show any change in the host framework ( Supplementary Fig. S12 ). In addition, solid-state 2 H NMR spectra of the deuterated zinc analogue of 1a -encapsulating PEG showed that the motion of the terephthalate ligand was almost unchanged and quiescent from −60 to −20 °C ( Supplementary Figs S13 and S14 ), suggesting no motional correlation between the host framework and PEG around the transition temperature. Thus, the host framework is not involved in the thermal transition process from the viewpoints of structure and molecular motion, and the transition observed in DSC indeed originates from the guest PEG chains. Detailed DSC analyses for 1a ⊃ PEG were carried out to gain insight into the transition behaviour of PEG within the channels. The effect of amount of PEG in the pore on the transition peak was examined by changing the ratios of PEG to 1a (PEG/ 1a =20–45 weight%), which revealed that the peak position and the transition heat for the confined PEG were fairly independent of the amount of PEG loaded in the channels ( Supplementary Fig. S15 ). This suggests that the PEG molecules prefer to form aggregated (bundled) structures in the 1-D channels rather than to be dispersed throughout the channels during the transition process [28] . In this system, interactions among PEG–PEG chains, such as hydrogen bonding, are still effective in the channels, resulting in the aggregation of PEG chains. Heating and cooling processes of DSC scans for 1a ⊃ PEG upon changing the scan speed were also investigated ( Supplementary Fig. S16 ). The exothermic peaks were found to move to lower temperatures with an increase in the cooling speed, which means a supercooling behaviour for PEG. In addition, the exothermic peaks obtained in the cooling process and the endothermic peaks in the heating process are accompanied by a significant hysteresis, indicating that this thermal behaviour is a first-order transition [29] . Although it might be inappropriate to use bulk concepts for defining the phase state of a substance confined in nanoscale pores, all of these results suggest that the transition found in this system can apparently be interpreted as a melting–freezing behaviour of PEG, where this is the first example of observing a thermal transition of polymers confined below the 1nm region. To understand the detailed transition behaviour of the confined PEG, we performed several experimental and theoretical analyses and showed that this thermal transition practically involves different mechanisms from the melting of bulk PEG. In the variable temperature infrared spectra of 1a ⊃ PEG, the bands corresponding to the conformation of PEG (around 915, 950, 1250 and 1,300 cm −1 ) showed a slight change from −80 to 0 °C, suggesting that the chain conformation is almost retained during the transition process ( Supplementary Fig. S9 ) [24] . This phenomenon is in contrast with the melting of PEG in the bulk state, where the transformation from bulk crystal to liquid is accompanied by a large conformational change of the PEG chains [24] , [30] . Kinetic analysis of the non-isothermal DSC process was performed using the Ozawa method to confirm the transition mechanism of PEG occurring in the confined geometry ( Supplementary Fig. S17 ) [31] . The analysis of PEG in the channels of 1a showed that the freezing of PEG molecules is constrained, and seems to be nearly a 1-D mechanism, whereas bulk PEG crystals grow with a higher dimensionality. In addition, we carried out canonical Monte Carlo (MC) simulations using the simple modelling approach of PCP frameworks [32] . The simulations were performed taking into consideration the chemical and physical parameters of 1a and PEG. 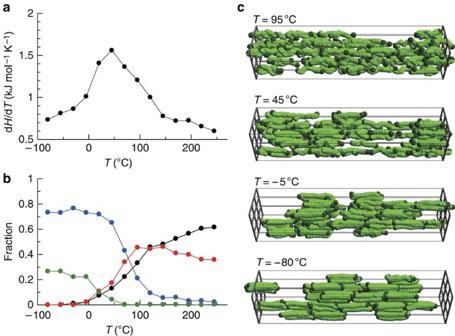Figure 3: Monte Carlo simulations for polymeric chain molecules confined in 1-D channels. (a) Calculated differential enthalpy profile on cooling of chain molecules confined in 1-D channels. (b) Temperature dependence of the number of associated chain molecules (monochain (black), dichain (red), trichain (blue) and tetrachain (green)) that belong to an assembly. (c) Snapshots of chain molecules in the confined 1-D space for different temperatures. Pore walls are not shown for clarity. The pseudoatoms at both ends of a chain molecule are shown in deep green, whereas others in light green. In Figure 3a , the differential enthalpy profile on cooling the chain molecules inside the 1-D channel shows a transition peak at 50 °C. As seen in Figure 3b , only monochains and dichains (assemblies of parallel-arranged two-chain molecules) exist at higher temperatures, whereas trichains and tetrachains become dominant at temperatures below 50 °C. Because the number of trichains and tetrachains increases rapidly with decreasing temperature from 100 to 0 °C, the transition peak is attributable to the stabilization arising from the formation of chain molecule assemblies. In addition, these trichains and tetrachains tend to localize and form a domain structure, which contrasts with the uniform distribution of molecules at higher temperatures ( Fig. 3c ). The interaction over pore walls seems relatively strong, bringing the isolated assemblies together to form the domain structure. Thus, our simulations demonstrate that the peak of the differential enthalpy would result from a transition between the distributed “liquid-like” state and the localized dense domain structure of chain assemblies. Figure 3: Monte Carlo simulations for polymeric chain molecules confined in 1-D channels. ( a ) Calculated differential enthalpy profile on cooling of chain molecules confined in 1-D channels. ( b ) Temperature dependence of the number of associated chain molecules (monochain (black), dichain (red), trichain (blue) and tetrachain (green)) that belong to an assembly. ( c ) Snapshots of chain molecules in the confined 1-D space for different temperatures. Pore walls are not shown for clarity. The pseudoatoms at both ends of a chain molecule are shown in deep green, whereas others in light green. Full size image Effect of pore characteristics on the thermal transition of PEG In the PCP materials [Cu 2 (L) 2 (ted)] n ( 1 ), precision control of the 1-D channel structures at the subnanometre size level can be attained by changing the dicarboxylate ligands L; thus, the effect of pore size on transition temperatures of PEG can be studied using 1a–e , with channel sizes from 0.4 to 1.1 nm ( Fig. 1 and Supplementary Fig. S1 ). In this system, the transition temperature of PEG confined in PCPs is denoted as T tr . As the pore size of 1 becomes larger, the number of PEG chains that can be aligned in the cross-section of the channels is expected to increase ( Supplementary Fig. S18 ). Direct inclusion of PEG into the host channels by polymer-melt processing successfully gave 1 ⊃ PEG composites ( Supplementary Figs S2–S5 ), and the guest PEG chains are encapsulated, with linear conformation with slightly distorted structures in the channels, similar to the case of 1a ( Supplementary Fig. S8 ). 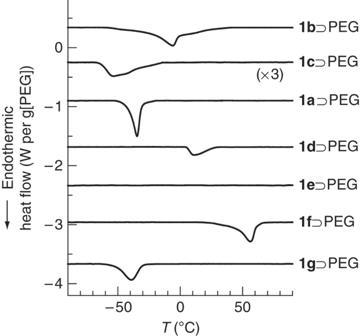Figure 4: DSC measurements of PEG confined in PCP pores. DSC heating curves of PEG (Mw=600) encapsulated in various PCP hosts1. The effect of pore size on the T tr was studied using DSC, as shown in Figure 4 . In the previous confined systems, transition temperatures of nanoconfined materials decrease as the confined spaces become narrower, which is explained by the Gibbs–Thomson equation based on classical thermodynamics [15] , [16] . However, this rule fails for micropores (<2 nm) because of the large heterogeneity of the confined materials and strong surface interactions, and the transition behaviours of confined materials finally disappear below their critical sizes [15] , [16] , [33] , [34] , [35] . In contrast, T tr of PEG was clearly detected even in the subnanometre channels of PCPs and showed a unique non-monotonic variation ( Fig. 4 ). As the pore size of 1 became narrower, T tr of the confined PEG decreased and reached the lowest value (−53 °C) in the system using 1c . However, further decreasing the pore size led to the increase in T tr of the confined PEG. It is of note that no endothermic peak was detected in the case of PEG in the smallest diameter pores ( 1e ), probably because of only single-chain accommodation in the channels. These unique thermal transition behaviours were also confirmed by the solid-state CP–MAS 13 C NMR measurements using non-magnetic zinc analogues of 1 and [Zn 2 (L) 2 ted] n ( 2a , L=terephthalate; 2d , L=1,4-naphthalenedicarboxylate; and 2e , L=9,10-anthracenedicarboxylate), as host matrices ( Fig. 5 ). The peaks corresponding to PEG chain accommodated in the channels were detected at around 70 p.p.m. in the spectrum [36] , [37] , [38] . In measurements of 2a ⊃ PEG and 2d ⊃ PEG with increasing temperature, steep decreases in linewidths of the peaks for PEG were observed around the T tr because of the thermal transition of PEG from a rigid state to a highly mobile state ( Fig. 5 and Supplementary Fig. S13 ) [39] . However, in the case of 2e ⊃ PEG, the peak for PEG showed a gradual decrease in the linewidths with increasing temperatures because of the lack of a cooperative transition of PEG in this host matrix ( Fig. 5 and Supplementary Fig. S13 ). Figure 4: DSC measurements of PEG confined in PCP pores. DSC heating curves of PEG ( M w =600) encapsulated in various PCP hosts 1 . 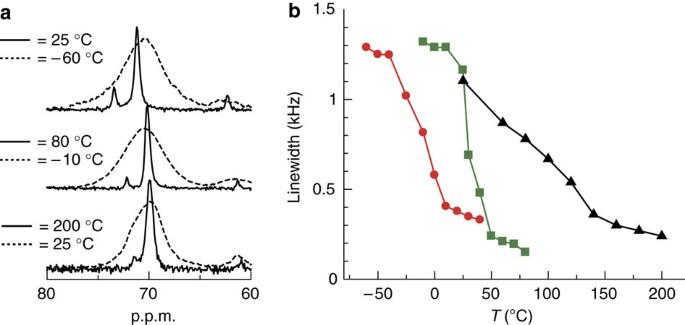Figure 5: Solid-state CP MAS13C NMR measurements for PCP–PEG composites. (a) CP MAS13C NMR spectrum of (top)2a⊃PEG, (middle)2d⊃PEG and (bottom)2e⊃PEG (Mwof PEG=600). At lower temperatures, all the spectra showed a broad peak at 70 p.p.m. corresponding to PEG inside the channels. These broad peaks became sharper with increase in the temperature, suggesting an increase in the mobility of PEG. Additional peaks detected around 72–74 and 61–62 p.p.m. were assignable to the terminal moieties of PEG. (b) Plots of full-width at half-maximum of the peak at 70 p.p.m. in the different temperature ranges (red=2a⊃PEG, green=2d⊃PEG and black=2e⊃PEG). Full size image Figure 5: Solid-state CP MAS 13 C NMR measurements for PCP–PEG composites. ( a ) CP MAS 13 C NMR spectrum of (top) 2a ⊃ PEG, (middle) 2d ⊃ PEG and (bottom) 2e ⊃ PEG ( M w of PEG=600). At lower temperatures, all the spectra showed a broad peak at 70 p.p.m. corresponding to PEG inside the channels. These broad peaks became sharper with increase in the temperature, suggesting an increase in the mobility of PEG. Additional peaks detected around 72–74 and 61–62 p.p.m. were assignable to the terminal moieties of PEG. ( b ) Plots of full-width at half-maximum of the peak at 70 p.p.m. in the different temperature ranges (red= 2a ⊃ PEG, green= 2d ⊃ PEG and black= 2e ⊃ PEG). Full size image The effect of pore surface functionality on the T tr of PEG was studied using 1d , 1f and 1g ( Fig. 1 and Supplementary Fig. S1 ). The porosities (pore sizes) of 1d , 1f and 1g are almost the same, as is confirmed by the X-ray crystal structure and guest adsorption analyses ( Supplementary Figs S18 and S19 ); however, their pore surface environments are quite different because of the functional groups, such as aromatic, methoxy and fluorinated moieties. To verify the various pore environments, heats of desorption for 2-ethoxyethanol, as a model compound for PEG, from the matrices of 1d , 1f and 1g were determined by DSC to be 57.9, 67.7 and 52.3 kJ mol −1 , respectively, which suggests the order of interaction of the guest PEG with the pore walls: 1f > 1d > 1g . These specific surface properties of the pores had significant roles in determining T tr of the confined PEG ( Fig. 4 ). The DSC scans of PEG included in the channels of 1d , 1f and 1g exhibited endothermic peaks at 20, 56 and −39 °C, respectively. It is of note that T tr of PEG in 1f was found to be higher than that of neat PEG (22 °C). Thus, the T tr of PEG in PCPs is finely controllable and becomes higher as the PEG–pore attractive interaction increases. Dependence of transition temperature on molecular weight of PEG A very striking result was obtained from a study of the effect of molecular weight of PEG in this system. In conventional bulk molecular systems, it is commonly observed that molecules with higher molecular weight show higher melting temperatures in the same family, for example, ethane, n -butane and n -octane melt at −183, −138 and −60 °C, respectively. Similarly, the melting temperature of neat PEG increases as the molecular weight of PEG increases. However, in stark contrast to the neat system, the transition of PEG confined in the channels of 1a exhibited the opposite molecular weight dependence: the higher the molecular weight of the PEG incorporated, the lower the observed T tr ( Fig. 6 ). 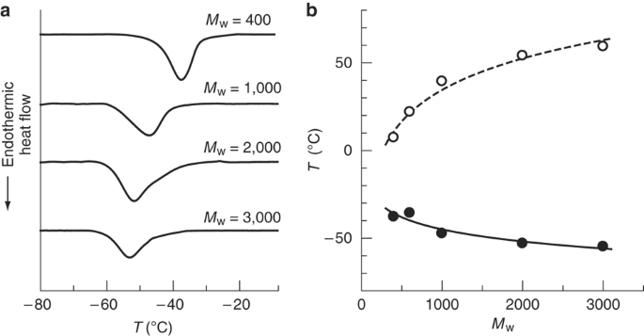Figure 6: Dependence ofTtron molecular weight of PEG. (a) DSC heating curves of PEGs with the different molecular weight incorporated in1a. (b) Molecular weight dependence of the melting temperatures of the bulk PEG (open circles) and theTtrs of PEG encapsulated in1a(filled circles;Mw/Mnof PEG used in this study was 1.02–1.06). Figure 6: Dependence of T tr on molecular weight of PEG. ( a ) DSC heating curves of PEGs with the different molecular weight incorporated in 1a . ( b ) Molecular weight dependence of the melting temperatures of the bulk PEG (open circles) and the T tr s of PEG encapsulated in 1a (filled circles; M w / M n of PEG used in this study was 1.02–1.06). Full size image The pore size and surface effects of our PCP system can be easily tailored at the subnanometre level, allowing systematic control of the transition behaviour of the confined PEG. For example, T tr of the confined PEG was found to be strongly dependent on the pore sizes of 1a–d and showed a unique non-monotonic variation ( Fig. 4 ). In this series of PCPs, the reduction in T tr is explained by the destabilization of the solid state in confined spaces [15] , [16] . The T tr elevation observed in narrower pores can be ascribed to the interactions of the guest polymers with hosts at the interface between them, and the interaction is expected to increase with a decrease in the pore size [10] , [15] , [16] , [35] . Such host–guest interactions cause a decrease in the PEG mobility to induce the solidification of PEG assembly. When PEG chains were incorporated in the channels of 1d , 1f and 1g with different surface functionalities, the T tr of confined PEG became higher with increase in the affinity ( 1g < 1d < 1f ) between the pores and PEG ( Fig. 4 ). Therefore, the molecular motion of PEG in the channels of PCPs can be determined by counterbalancing the size effect and the pore–guest interaction [10] , leading to the remarkable variation in T tr of the confined PEG. The disappearance of T tr for PEG in the narrowest pores of 1e is probably because of the single-chain accommodation. Because the thermal transition behaviour is such a molecularly cooperative phenomenon, a single PEG chain cannot show such a transition, resulting in the suppression of the DSC peak. An unprecedented molecular weight dependence of the polymer thermal transition was also observed in our PCP pores. In conventional bulk systems, molecules with higher molecular weight usually show higher thermal transition temperatures in the same family. In contrast, our confinement system showed a remarkable decrease in T tr of PEG with an increase in its molecular weight in the channels of 1a ( Fig. 6 ). This unusual behaviour can be explained by the fact that the solid-like state of PEG chains is destabilized in the channels. In this situation, the effect of destabilization per one PEG chain would be more enhanced when longer chains are incorporated in 1a . Understanding the behaviour of ultrathin polymer assemblies at the subnanometre level is important because of their potential application as nanosized transporters, lubricants and connectors in molecular-based devices. However, it remains a major challenge to understand the confinement effect of polymer materials and to control their properties in the subnanometre regime. By utilizing regular PCP channels as host matrices, our results have led to significant progress in understanding thermal transitions in confined polymer materials. We believe that our results will provide new insights into polymer transition behavior in nanoconfined geometries. Materials All reagents and chemicals were obtained from commercial sources unless otherwise stated. PEG samples were used as received and their molecular weight distributions ( M w / M n ) were 1.02–1.06, as determined by gel permeation chromatography using universal calibration with PEG standards. Activated carbon fibre ACF A-5 was kindly supplied by Osaka Gas. The host PCP compounds [Cu 2 (L) 2 ted] n ( 1 ) and their zinc analogues, [Zn 2 (L) 2 ted] n ( 2 ), were prepared by previously described methods [23] , [40] , [41] , [42] , [43] . Partially deuterated PCPs were synthesized using terephthalate- d 4 and 1,4-naphthalenedicarboxylate- d 6 [44] . Introduction of PEG into PCPs The host–guest composites of 1 ⊃ PEG were prepared by direct encapsulations of PEG into host matrices [10] , [12] . The inclusion ratios of PEG to 1 were adjusted not to exceed the completely filled amounts in the nanochannels, which depends on the porosities of 1 . Typical incorporation amounts of PEG in 1 (weight of PEG/weight of 1 ) are as follows: 1a , 0.40; 1b , 0.67; 1c , 0.40; 1d , 0.25; 1e , 0.25; 1f , 0.25; 1g , 0.25. Treatment of PCPs with excess amounts of PEG results in the appearance of a DSC peak corresponding to melting of bulk PEG, because excess PEG exists outside host crystals ( Supplementary Fig. S15 ). The general incorporation procedure is as follows: a host compound 1a (100 mg) was dried by evacuation at 130 °C for 5 h. Subsequently, this was immersed in a CH 3 CN solution (1 ml) of PEG (40 mg, M w =600) at room temperature. To incorporate the PEG into the nanochannels, CH 3 CN was completely removed by evacuation at the elevated temperature of 90 °C (above the T m of neat PEG) for 12 h to obtain a powdery composite 1a ⊃ PEG. Elemental analysis (%) for 1a ⊃ PEG (40 weight%). Found: C, 47.99; H, 5.17; N, 3.14%. Calcd. for C 32.0 H 40.8 N 2.0 O 13.4 Cu 2.0 : C, 48.40; H, 5.17; N, 3.52. MD simulation and density functional theory calculation To localize the crystallographically equivalent atomic sites in the X-ray structure of 1a , the framework of 1a was fully optimized under the three-dimensional periodic boundary conditions, with the Perdew–Wang 1991 (PW91) functional parameters within the generalized gradient approximation. Employing the ultrasoft pseudopotential method, the (2 × 2 × 3) Monkhorst–Pack k -point mesh was used to sample the Brillouin zone. The kinetic energy cutoff for the plane waves was set to 400 eV. The optimized fractional coordinates of all atom positions per a unit cell, cell lengths and angles for the optimized structure of 1a were almost the same as those obtained from the X-ray diffraction experiment. PEG 14mer ( M w =634.7) was modelled according to the crystal structure [25] and was introduced into the optimized framework of 1a . Energy minimization of the model was initially done by applying the universal force field. To duplicate the experimental condition of annealing, the canonical (constant particle number N, volume V, and temperature T)–MD simulation was initially conducted by heating the model up to 400 K, followed by the cooling NVT–MD simulation down to 200 K. The product run of equilibrium MD simulation was then executed for 1,500 ps. All the MD simulations were done with a time step of 1 fs, the host framework being fixed. To obtain the infrared spectra, by utilizing Gaussian03, we performed vibrational frequency analysis for both four single PEG 14mers in the channel of 1a and a 7mer in crystal at the PW91PW91/6-31G(d) level of theory. Canonical MC simulation Following the simple modelling approach of PCP frameworks [32] , the host 1-D channel was composed of smooth walls placed at an equal interval so that they construct 1-D channels with square cross-section. The chain molecule was also simplified and modelled on n -alkane using the united atom model that treats CH 3 and CH 2 as single interaction centres (pseudoatoms). The bond length between pseudoatoms was fixed and the bending and torsional potentials were considered. The potential parameters were given on the basis of the transferable potential for phase equilibria model [45] . The number of pseudoatoms in a single-chain molecule was set to be 24. To model the 1a ⊃ PEG system with less interaction between the host PCP and the guest chain molecule, the hard-wall potential was assumed between chain molecules and the pore walls. The simulation unit cell was composed of nine (3 × 3) channels. The center-to-center distance between walls, the wall thickness and the cell length in the channel direction were respectively set to be 3.3 σ , 1.2 σ and 50 σ , where σ is the size parameter of the pseudoatom CH 2 . With this pore size, four chain molecules can be at most aligned in parallel, which is consistent with the combination of 1a and PEG. The periodic boundary condition was applied for all directions. The simulations of the chain molecules on cooling were performed in a canonical ensemble, which corresponds to the experimental procedure of the DSC analysis conducted after the PEG inclusion into the host PCP. To achieve efficient sampling of the simulations of long chain alkanes, the configurational bias MC technique was used [46] . In this technique, MC moves include translation, rotation and re-growing parts of a molecule. The number of chain molecules was 90 in the simulation box. The length of a simulation run was at least 5.4 million MC steps. Near the structural transition, 36 million MC steps were performed. The last configuration of a run was used as the initial configuration of the next run with a lower temperature. The enthalpy of the system was given by the following equation: where the bracket indicates the ensemble average; U , the total internal energy per molecule; p , the external pressure; V pore , the volume per molecule. The second term pV pore is assumed to be negligible compared with the first term. The total internal energy U is generally given by where U K is kinetic energy; U CC and U CW , the chain–chain (CC) and the chain–wall (CW) contributions; N , the number of chain molecules in the system; U intra , the intramolecular contribution owing to the bending, torsional and non-bonding interactions. Note that U CW is zero in the present condition because the hard-wall potential is assumed. The first term U K is given by 1/2 k B T per degree of freedom of a chain molecule, where k B is the Boltzmann constant and T is the temperature. The degree of freedom in the 1-D channel is expected to be smaller than that in bulk because the confined space suppresses the motion of chain molecules, although the exact value is difficult to estimate. However, the discussion on the differential enthalpy profile d H /d T is possible without the U K term, because d U K /d T is assumed to be constant and just shift the profile in parallel. We accordingly calculated the second and third terms in the above equation for the enthalpy calculation. The calculated enthalpy was numerically differentiated to obtain the differential enthalpy. To judge whether molecules i and j form an assembly, the distance r ij averaged over all combinations of two pseudoatoms chosen from different molecules i and j was calculated. The two molecules were considered to belong to the same aggregate when the averaged distance r ij was <3.7 σ . Measurements XRPD data were collected on a Rigaku RINT 2000 Ultima diffractometer with Cu Kα radiation. SEM measurement was performed using a Hitachi S-3000N at an accelerating voltage of 5 kV. Samples were put on a conducting carbon tape attached by SEM grid, and then coated with platinum. Particle size distribution was obtained by Horiba Partica LA-950 laser diffraction particle size analyser. Elemental analysis was performed on a Flash EA 1112 series (Thermo Finnigan instrument). The adsorption isotherms of nitrogen at 77 K were measured with a Quantachrome Autosorb-1 volumetric adsorption instrument. Nitrogen gas of high purity (99.9999%) was used. Before the adsorption measurements, the sample was treated under reduced pressure (<10 −2 Pa) at 373 K for 5 h. DSC analysis was carried out with a Mettler Toledo DSC822e/200 under N 2 atmosphere. The weight of the samples ranged from 4 to 6 mg. All the measurements were preceded by heating of the samples to 120 °C at a heating rate of 10 °C min −1 to remove the thermal history. Then, the samples were cooled down to −100 °C at a cooling rate of 10 °C min −1 and were subsequently heated at a heating rate of 10 °C min −1 to obtain the heating curves. The micro-Raman measurements were carried out at room temperature using the Raman spectrometer HORIBA Jobin Yvon LabRam HR800, equipped with an Olympus confocal optical microscope. The excitation light source was a semiconductor laser of 784.4 nm wavelength and the beam was focused onto the sample using an optical microscope (×100 magnification), which allowed us to focus the laser beam with a 1 μm lateral resolution and an axial depth resolution of about 3 μm. Infrared spectra were measured using KBr disc with a PERKIN ELEMER Spectrum BX FT-infrared system. Variable temperature infrared spectra were obtained with a Thermo Electron Nicolet 6700 FT-infrared spectrometer. The samples were placed in a Linkam LK-600 hot stage under N 2 atmosphere. Thermogravimetric analysis was performed at 10 K min −1 using a Rigaku Instrument Thermo plus TG 8120 in a nitrogen atmosphere. CPMAS 13 C NMR was measured by JEOL JNM-LA300WB spectrometer operated at 75.6 MHz. 2 H NMR spectra were measured by a Varian Chemagnetics CMX-300 spectrometer at 45.8 MHz with a quadrupole pulse sequence. Frequency-switched Lee–Goldburg (LG) heteronuclear 1 H– 13 C correlation spectra were measured with an LG period of 11.4 μs coupled with the magic angle spinning of 8–12 kHz on a Bruker Avance 400 wide bore instrument. Quadrature detection in t 1 was achieved by a time proportional phase increments method. Carbon signals were acquired during t 2 under proton decoupling applying a two-pulse phase modulation scheme. How to cite this article: Uemura, T. et al . Unveiling thermal transitions of polymers in subnanometre pores. Nat. Commun. 1:83 doi: 10.1038/ncomms1091 (2010).